Quantitative experimental determination of site-specific magnetic structures by transmitted electrons With rapid progress in the fields of nanomagnetism, multiferroics and spintronics, a method to characterize local magnetic structure information of the nanostructures is of essential importance for understanding and designing the magnetic materials on a nanometre scale. However, the site-specific magnetic structure determination from a nanoscale region in complex materials is challenging. Electron energy-loss magnetic chiral dichroism (EMCD) [1] technique was invented as a new route for detecting the magnetic signals using the transmitted electron beam with a reported high spatial resolution [2] . The capability of EMCD in quantitatively solving magnetic structures is fundamentally dependent on the strong dynamical diffraction effects of fast electrons [3] , [4] . The dynamical diffraction effects of fast electrons had been constructively applied using the technique of atom-location channelling enhanced micro-analysis [5] , [6] , [7] , [8] , especially the energy loss by channelled electrons technique [9] , to obtain the site-specific information, such as element contents, valence states and electronic configurations. Some theoretical EMCD calculations [10] , [11] and experimental work [12] discussed about the site specificity of the EMCD signals. In this work, we experimentally demonstrate how we develop the site-specific EMCD method by adjusting dynamical diffraction conditions to modulate the magnetic circular dichroism (MCD) signals at non-equivalent crystallographic sites, and further using dynamical diffraction calculations to extract the site-specific MCD spectra with quantitative site-specific magnetic structure information obtained in an example of NiFe 2 O 4 (NFO). Compared with previous EMCD works on the detection and analysis of ferromagnetic signals [13] , [14] , in this work we develop the site-specific EMCD method as a unique technique, which is capable of quantitatively solving the unknown magnetic structures of the materials with non-equivalent crystallographic sites in a nanoscale level with a high site specificity. It is the first work to experimentally demonstrate that the transmitted electron source can be used to quantitatively determine magnetic structure in complex materials. Sample information Here, we studied the NFO single crystal in a nanometre-scale composite film [15] , [16] . The low-magnification transmission electron microscope (TEM) image of the composite film and the selected area electron diffraction patterns of an NFO nanopillar in [110] zone axis are shown in Fig. 1 . The NFO crystal has an inverse spinel structure and ferrimagnetic structure, which is written as (Fe 3+ ↓) A (Ni 2+ ↑ Fe 3+ ↑) B O 4 at its nominal stoichiometric ratio [6] , [15] . The ‘A’ and ‘B’ notations represent tetrahedral sites (tet) with downward-direction (↓) magnetic moments and octahedral sites (oct) with upward-direction (↑) magnetic moments, respectively. Owing to the magnetic field of ∼ 2 T of the objective lens exerted on the specimen, the upward direction (↑) refers to the direction parallel to the magnetic field, while the downward direction (↓) refers to the direction anti-parallel to the magnetic field. Other necessary information about the sample is given in the section of Methods. 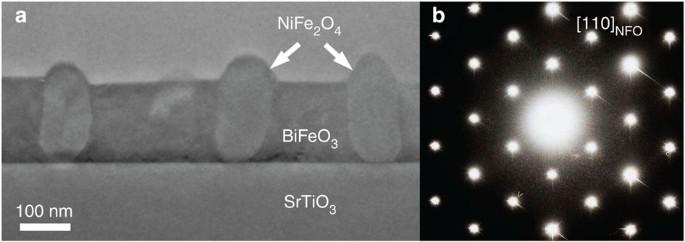Figure 1: Transmission electron microscopy (TEM) image and selected area electron diffraction (SAED) patterns of cross-sectional composite films. (a) Low-magnification TEM image for cross-section sample of hetero-epitaxial composite thin films formed by perovskite BFO and spinel NFO on the substrate of SrTiO3. (b) SAED patterns for one NFO crystal nanopillar tilted to the [110] zone axis. Figure 1: Transmission electron microscopy (TEM) image and selected area electron diffraction (SAED) patterns of cross-sectional composite films. ( a ) Low-magnification TEM image for cross-section sample of hetero-epitaxial composite thin films formed by perovskite BFO and spinel NFO on the substrate of SrTiO 3 . ( b ) SAED patterns for one NFO crystal nanopillar tilted to the [110] zone axis. Full size image Dynamical diffraction effects on EMCD signals The dynamical diffraction effects of fast electrons are mainly influenced by the incident and outgoing electron orientations, which change the distributions of incident and reciprocal waves, respectively [17] , [18] , and sample thickness is another key factor [11] , [19] . The dynamical diffraction conditions for fast electrons have essential impacts on the EMCD spectra, that is, to modulate the weights of MCD signals from different atoms at different crystallographic sites in the sample. The influences of different incident electron orientations on EMCD signals are compared in Fig. 2a . Twenty-nine nanometer-thick NFO crystal is oriented to the three-beam case with (004) systematic reflections excited (cf. Fig. 2a ) and with (22̄0) systematic reflections excited (cf. Fig. 2b ). The electron energy-loss spectroscopy (EELS) spectra were acquired at + and − positions for EMCD measurements [1] . In Fig. 2a , extremely strong EMCD signals (about 33% difference for Fe and 42% for Ni) were observed [13] , [14] , [20] , which are critical for further quantitative analysis of magnetic structures. Here, we define that an EMCD signal of Fe or Ni has a ‘L3−L2+’ sign in case that it is negative on L 3 edge and positive on L 2 edge, while the contrary situation corresponds to a ‘L3+L2−’ sign. Comparing the EMCD signals in Fig. 2 , the ‘L3−L2+’ sign for Fe in Fig. 2a is opposite to the ‘L3+L2−’ sign for Fe in Fig. 2b , while the ‘L3−L2+’ sign for Ni in Fig. 2b is the same as that of Ni in Fig. 2a . The data points of the original EELS spectra in Fig. 2 are shown in Supplementary Fig. S1 . 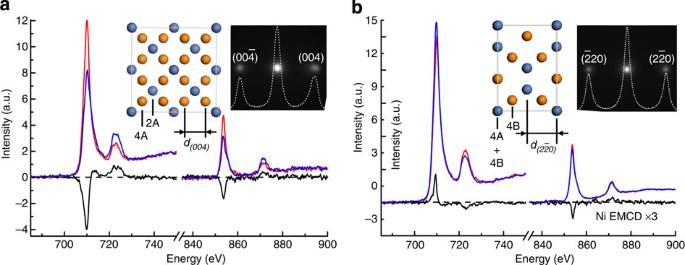Figure 2: Electron energy-loss magnetic chiral dichroism (EMCD) spectra measured in three-beam conditions with (004)/(22̄0) systematic reflections excited. (a) EMCD measurement on 29-nm-thick NFO sample in three-beam conditions with (004) systematic reflections excited where 2A (blue), 4B (orange), 2A, 4B… crystal planes are parallel to the incident beam as shown in the inset of crystal lattice. The inset of diffraction plane shows the symmetrical excited diffraction spots and its intensity profile in experiment. The spectra are Fe and NiL2,3edges taken on two chiral positions ‘+’ and ‘−’ (shown in red and blue, respectively), and EMCD signal (the difference spectra, shown in black colour) for Fe and NiL2,3edges. (b) EMCD measurement on 29-nm-thick NFO sample in three-beam conditions with (22̄0) systematic rows excited where 4A+4B, 4B, 4A+4B, 4B… crystal planes are parallel to incident beam. FeL2,3edges and NiL2,3edges taken from ‘+’ and ‘−’ positions, and the corresponding EMCD spectra. Figure 2: Electron energy-loss magnetic chiral dichroism (EMCD) spectra measured in three-beam conditions with (004)/(22̄0) systematic reflections excited. ( a ) EMCD measurement on 29-nm-thick NFO sample in three-beam conditions with (004) systematic reflections excited where 2A (blue), 4B (orange), 2A, 4B… crystal planes are parallel to the incident beam as shown in the inset of crystal lattice. The inset of diffraction plane shows the symmetrical excited diffraction spots and its intensity profile in experiment. The spectra are Fe and Ni L 2,3 edges taken on two chiral positions ‘+’ and ‘−’ (shown in red and blue, respectively), and EMCD signal (the difference spectra, shown in black colour) for Fe and Ni L 2,3 edges. ( b ) EMCD measurement on 29-nm-thick NFO sample in three-beam conditions with (22̄0) systematic rows excited where 4A+4B, 4B, 4A+4B, 4B… crystal planes are parallel to incident beam. Fe L 2,3 edges and Ni L 2,3 edges taken from ‘+’ and ‘−’ positions, and the corresponding EMCD spectra. Full size image The changes in signs for the EMCD signals can be qualitatively explained by dynamical diffraction effects. In the three-beam case with (004) systematic rows excited, alternating (008) octahedral and tetrahedral planes (with 4B and 2A atoms, respectively, on each plane in a unit cell) are parallel to incident electrons as shown in the inset of Fig. 2a . The 4B planes with deeper potential energy wells are channelled along by electrons, and the MCD signals from 4B planes are enhanced. The Fe and Ni EMCD signals with ‘L3−L2+’ sign reflect the dominating excitation of 2Fe 3+ ↑ and 2Ni 2+ ↑ atoms on 4B planes. In the three-beam case with (22̄0) systematic rows excited, alternating 4A+4B and 4B planes are parallel to incident electrons (cf. inset of Fig. 2b ). The enhanced 4A+4B (4Fe 3+ ↓+2Fe 3+ ↑+2Ni 2+ ↑) planes with the dominating contributions from Fe 3+ ↓ and Ni 2+ ↑ atoms lead to ‘L3+L2−’ sign Fe EMCD signal and ‘L3−L2+’ sign Ni EMCD signal. It is concluded that the different relative weights of MCD signals from octahedral (B) sites and tetrahedral (A) sites at the two dynamical diffraction conditions lead to the opposite signs for Fe EMCD spectra in Fig. 2a . Moreover, the weights of MCD signals from octahedral sites and tetrahedral sites can also be modulated by varying the outgoing electron orientations. For example, with (004) systematic reflections excited, the incident angle θ in,004 (angle between incident electrons and (004) crystal planes) for a 42-nm-thick NFO is tilted to be 2 θ B ( θ B is the Bragg angle for NFO (004) crystal planes) with tetrahedral sites enhanced for incident waves as shown in Fig. 3a . The EMCD spectra at different outgoing angles are investigated by locating the + and − detectors in five pairs of positions as shown in Fig. 3b , corresponding to outgoing angles of 2 θ B , θ B , 0, − θ B , −2 θ B . For reciprocal waves, it tends to enhance different sites at different outgoing angles, and the signs of experimental EMCD spectra (cf. in Fig. 3c ) are observed changing with the outgoing angles. There shows no EMCD signal at outgoing angle of 2θ B . The data points of the original EELS spectra in Fig. 3 are shown in Supplementary Fig. S2 . The EMCD signal distribution on the diffraction plane for the above dynamical diffraction conditions was simulated depending on the theoretical dynamical diffraction calculation methods ( Supplementary Fig. S3 , Supplementary Discussion and Supplementary Methods ), which was consistent with the signs of the experimental EMCD signals at different outgoing angles. The EMCD signals also vary with sample thickness owing to dynamical diffraction effects [11] , [20] (see Supplementary Fig. S4 ). The sample with uniform and optimized thickness is selected to obtain EMCD spectra with high signal-to-noise ratio. To accurately measure thickness in a thin area via low-loss EELS [21] , which is essential for the EMCD quantitative analysis, the mean free path [21] is calibrated in the thick NFO area, where the thickness is precisely determined using the convergent beam electron diffraction method. The high S/N ratios in our EMCD experiments are attributed to the performance of the microscope, the high site specificity of EMCD signals for NFO and the optimized dynamical diffraction conditions ( Supplementary Discussion ). 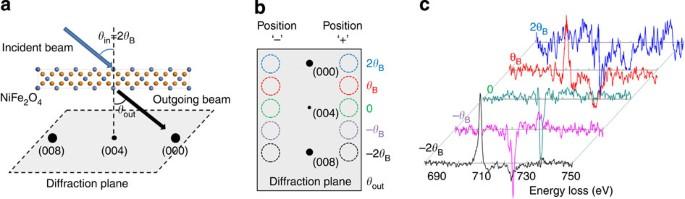Figure 3: Electron energy-loss magnetic chiral dichroism (EMCD) spectra of Fe with the incident angleθin,004=2θBfor (004) systematic reflections at five different outgoing angles. A 42-nm-thick NFO sample was used. (a) The incident angleθin,004=2θBfor (004) systematic reflections was used. The sketch of incident beam, outgoing beam and the diffraction patterns. (b) The ‘+’ and ‘−’ entrance aperture was located at five pairs of positions corresponding to different outgoing angles of 2θB,θB, 0, −θB, −2θB, respectively. At a specific outgoing angle, ‘+’ and ‘–’ positions for EMCD measurement are chosen to be in mirror symmetry with respect to (004) reflection with a perpendicular distance of 0.8g004. (c) Corresponding EMCD spectra of Fe taken on the five outgoing angles. The EMCD signal of oct Fe is dominating at outgoing angles of 0 and −θBleading to ‘L3−L2+’ EMCD spectra, while the EMCD signal of tet Fe is dominating at outgoing angles ofθBand −2θBleading to ‘L3+L2−’ EMCD spectra. Figure 3: Electron energy-loss magnetic chiral dichroism (EMCD) spectra of Fe with the incident angle θ in,004 =2 θ B for (004) systematic reflections at five different outgoing angles. A 42-nm-thick NFO sample was used. ( a ) The incident angle θ in,004 =2 θ B for (004) systematic reflections was used. The sketch of incident beam, outgoing beam and the diffraction patterns. ( b ) The ‘+’ and ‘−’ entrance aperture was located at five pairs of positions corresponding to different outgoing angles of 2 θ B , θ B , 0, − θ B , −2 θ B , respectively. At a specific outgoing angle, ‘+’ and ‘–’ positions for EMCD measurement are chosen to be in mirror symmetry with respect to (004) reflection with a perpendicular distance of 0.8g 004 . ( c ) Corresponding EMCD spectra of Fe taken on the five outgoing angles. The EMCD signal of oct Fe is dominating at outgoing angles of 0 and − θ B leading to ‘L3−L2+’ EMCD spectra, while the EMCD signal of tet Fe is dominating at outgoing angles of θ B and −2 θ B leading to ‘L3+L2−’ EMCD spectra. Full size image Determination of magnetic structure information In the following sections, we will demonstrate how to solve the magnetic structure in NFO by site-specific EMCD and testify its validity in determining magnetic structure information by comparing with the results by theoretical calculations and other experimental techniques. To quantitatively distinguish the contributions of EMCD signals from atoms at oct and tet sites for further magnetic structure determination, dynamical diffraction calculations based on the theoretical framework [10] , [19] , [22] , [23] were performed ( Supplementary Methods ). Generally, the EMCD spectrum at a certain dynamical diffraction condition can be written as: where μ + and μ − are similar to the X-ray absorption spectra for incident photons with left and right circular polarizations [10] , respectively (see the definitions of μ + and μ − in Supplementary Methods ), and ( μ + − μ − ) represent the pure MCD spectra from atoms of oct Fe, tet Fe and oct Ni. The coefficients of a for octahedral sites and b for tetrahedral sites can be theoretically determined based on the crystallographic structure information of the material and the dynamical diffraction conditions ( Supplementary Methods ). The coefficients of a and b vary with dynamical diffraction conditions corresponding to different weights of MCD spectra from the atoms at different sites. It is calculated that the ratio of a (oct) to b (tet) for NFO in Fig. 2a is 1:−0.44 ( Supplementary Fig. S5 ), indicating that the MCD spectra from both oct Fe and tet Fe positively contribute to the strong experimental ‘L3−L2+’ sign Fe EMCD signal. In Fig. 2b , the ratio of a to b is 0.25:1, ( Supplementary Fig. S6 ) implying that the ‘L3+L2−’ sign EMCD signal of Fe mainly arises from the dominating MCD signal from tet Fe. The strong EMCD spectra in Fig. 2 are attributed to the enhancement effects under these dynamical diffraction conditions. Based on theoretically calculated coefficients of a and b , the site-specific MCD spectra of ( μ + − μ − ) oct,Fe , ( μ + − μ − ) tet,Fe and ( μ + − μ − ) oct,Ni are extracted from a series of experimental EMCD spectra at different dynamical diffraction conditions via statistical method of least square fitting that achieves the minimal residual errors, as shown in Fig. 4 ( Supplementary Fig. S7 and Supplementary Methods ). As a comparison, the site-specific MCD spectra cannot be experimentally obtained from X-ray magnetic circular dichroism (XMCD) except by simulating the spectra via multiplet calculations [24] . Even if at the beginning we knew nothing about the magnetic structure of NFO, the site-specific MCD spectra can give a clear demonstration of the ferrimagnetic structure of NFO, as the coefficients a and b are just calculated out using the knowledge of crystallographic structure information and dynamical diffraction condition. The general features of site-specific EMCD spectra are consistent with the previous simulated MCD spectra of oct Fe and tet Fe via multiplet calculations [24] , [25] . A possible energy shift of 0.4 eV between EMCD peaks of oct Fe and tet Fe in Fig. 4 is a reflection of the chemical shift for different site symmetries, which agrees with the simulated value [25] . 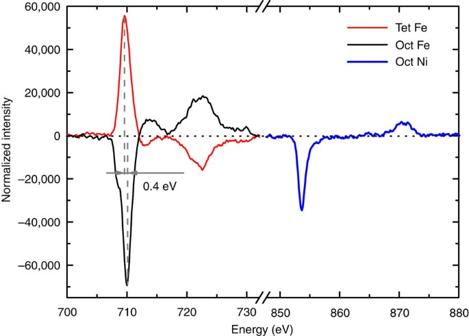Figure 4: Extracted site-specific magnetic circular dichroism pure spectra for oct Fe, oct Ni and tet Fe. A possible energy shift of 0.4 eV between oct Fe peak and tet Fe peak is a reflection of the chemical shift for different site symmetries. Figure 4: Extracted site-specific magnetic circular dichroism pure spectra for oct Fe, oct Ni and tet Fe. A possible energy shift of 0.4 eV between oct Fe peak and tet Fe peak is a reflection of the chemical shift for different site symmetries. Full size image Using the sum rules [4] , [11] , [26] , [27] , which allow a quantitative assessment of spin and orbital magnetic moments from the site-specific MCD spectra ( Supplementary Methods ), we further calculate the site-specific magnetic moments as shown in Table 1 . Compared with the results obtained by XMCD, neutron diffraction and first-principle calculation [20] , [28] , [29] , [30] , site-specific EMCD method shows the unique capability of solving magnetic structures experimentally and simultaneously achieving very comprehensive magnetic information. The orbital to spin magnetic moment ratios ( m L /m S ratios) for oct Fe and tet Fe are first reported, which are hardly acquired via other techniques. The m L /m S ratio for oct Ni measured by EMCD is close to that measured by XMCD [20] . It is the first time to use EMCD method to determine site-specific total magnetic moments (the sum of spin and orbital magnetic moments). The obtained site-specific total magnetic moment values are somewhat smaller but comparable with those measured by neutron diffraction and first-principle calculations. Besides, total magnetic moment in a unit cell of NFO by EMCD is close to that by macroscopic magnetic measurement [31] . The errors for the site-specific magnetic values are discussed in detail in Supplementary Table S1 and Supplementary Discussion . Table 1 Magnetic information for NiFe 2 O 4 via site-specific EMCD compared with that obtained from other techniques. Full size table Compared with other magnetic-characterization techniques, such as XMCD and neutron diffraction [30] , [32] , site-specific EMCD method has its unique advantages. XMCD lacks the ability of distinguishing magnetic contributions from different atomic sites. Neutron diffraction is difficult to distinguish magnetic contributions from atoms of different elements with close atomic form factor randomly distributed in a same site, and its spatial resolution is rather limited. In comparison, as shown in this work, site-specific EMCD method can achieve site-specific and element-specific magnetic information, as well as distinguish the orbital and spin magnetic moments in a nanoscale level, which displays its unique values. Generally, this work opens the door to quantitatively determine the site-specific magnetic structures for a wide range of magnetic materials in a nanoscale level using fast electrons. In the method of site-specific EMCD, dynamical diffraction effects of electrons are constructively used for tuning the site specificity through changing the Bloch wave fields, and considerably improve the EMCD signals. In the case of NFO, site-specific (oct Fe, tet Fe and oct Ni) total magnetic moments and m L /m S ratios were semiquantitatively and quantitatively, respectively, determined. The m L /m S ratios for oct Fe and tet Fe are for the first time reported here. It is first demonstrated that the transmitted electron source is capable to quantitatively determining magnetic structure in complex materials. Given the ability of quantitatively determining magnetic structures with comprehensive magnetic information in a nanometre-scale region, site-specific EMCD may benefit much to the research and application of magnetic materials as a unique magnetic-characterization tool. Sample preparation The sample in our experiment is a cross-section sample of hetero-epitaxial composite thin film formed by perovskite BiFeO 3 (BFO) and spinel NFO [15] , [16] . The low-magnification morphology image is shown in Fig. 1a . The composite thin film was grown by pulsed laser deposition at 700 °C on (001)-SrTiO 3 single-crystal substrate [15] . The ferrimagnetic NFO and antiferromagnetic BFO single-crystal nanopillars with the size of about 100 nm grow perpendicular to the substrate. Using high-resolution transmission electron microscopy and selected area electron diffraction, it is indicated that the NFO and BFO nanopillars not only grow epitaxial to the substrate in [001] orientation but also grow epitaxial to each other with the interface between them lying in the {110} orientation. When the NFO nanopillar is tilted to the [110] zone axis, (22̄0) and (002) reflections perpendicular to each other are excited in the diffraction plane, as shown in Fig. 1b . In the EMCD measurements, (22̄0) or (004) systematic reflections are, respectively, excited. BFO has a rhombohedrally distorted perovskite structure with antiferromagnetic magnetic structure, and exhibit weak ferromagnetism owing to a canted spin structure [33] . NFO has an inverse spinel structure. In spinel crystallography, NFO can be written as (Fe 3+ ) A (Ni 2+ Fe 3+ ) B O 4 in its nominal stoichiometric ratio. NFO is nearly a complete inverse spinel in that most of the Ni atoms occupy the octahedral sites, with δ ≈0.01 in the formula (Fe 1−δ Ni δ ) A (Fe 1+δ Ni 1−δ ) B O 4 [34] (ref. 34). Therefore, we do the calculation under the assumption that NFO is a complete inverse spinel with an error <1%. The energy dispersive spectroscopy measurements under non-channelling conditions show that the atomic ratio between Ni and Fe in our sample is 1:2. Acquisition of EMCD spectra The EELS and EMCD experiments were performed using a post-column Gatan Tridium system attached to the FEI Titan 80–300 TEM with Cs corrector, operating at 300 kV with an energy resolution of about 0.7 eV. The objective lens exerted a magnetic field of ∼ 2T on the specimen, whose magnetization is therefore saturated. In the EMCD measurements, nearly parallel beam (convergent angle <0.5 mrad) with the probe size of around 50 nm in diameter was used to illuminate the region inside an individual NFO nanopillar with uniform thickness. The specimen was tilted to the desired dynamical diffraction conditions ( Supplementary Fig. S8 and Supplementary Methods ). The incident conditions were precisely determined as shown in Supplementary Materials . The outgoing conditions were determined by the relative positions of diffraction spots to the entrance aperture, and the collection angle is about 4 mrad. The error in aperture position at diffraction plane is about 0.05 mrad and negligible owing to the strict geometrical construction. The data processing of the EELS spectra, including background subtraction from the pre-edge area, normalization by the post-edge area and Fourier-ratio deconvolution [35] using a zero-loss modifier function in Digital Micrograph, is discussed in detail in Supplementary Fig. S9 and Supplementary Methods . Calculations To obtain the dynamical coefficients for EMCD, the bw software [23] and the home-made codes were used based on the theoretical calculation frame [10] , [19] . The site-specific MCD spectra were extracted by least square fitting method from a series of EMCD spectra with the minimal residual errors for different dynamical diffraction conditions. Based on sum rules for MCD spectra, magnetic values are calculated for each atom in NFO [26] , [27] . Calculations of the magnetic structure of NFO were carried out using the projector augmented-wave method [36] within the density functional theory, as implemented in the VASP code [37] . Detailed calculation descriptions and error analysis can be found in Supplementary Methods . How to cite this article: Wang, Z.Q. et al . Quantitative experimental determination of site-specific magnetic structures by transmitted electrons. Nat. Commun. 4:1395 doi: 10.1038/ncomms2323 (2013).